Visualization and targeted disruption of protein interactions in living cells Protein–protein interactions are the basis of all processes in living cells, but most studies of these interactions rely on biochemical in vitro assays. Here we present a simple and versatile fluorescent-three-hybrid (F3H) strategy to visualize and target protein–protein interactions. A high-affinity nanobody anchors a GFP-fusion protein of interest at a defined cellular structure and the enrichment of red-labelled interacting proteins is measured at these sites. With this approach, we visualize the p53–HDM2 interaction in living cells and directly monitor the disruption of this interaction by Nutlin 3, a drug developed to boost p53 activity in cancer therapy. We further use this approach to develop a cell-permeable vector that releases a highly specific peptide disrupting the p53 and HDM2 interaction. The availability of multiple anchor sites and the simple optical readout of this nanobody-based capture assay enable systematic and versatile analyses of protein–protein interactions in practically any cell type and species. Great effort has been invested in the development of methods to identify protein interactions and screen for drugs that target specific protein–protein interactions. Although several useful in vitro methods have been developed, most of these assays disregard the innate complexity of living cells. In a live cell, protein–protein interactions are subjected to many influences such as subcellular localization, competitive interaction with other cellular factors and post-translational modifications. Drugs are usually screened in vitro in a very controlled and artificial environment. However, to work in vivo , the drugs must cross the cell plasma membrane and then reach their target protein in the respective subcellular compartments. Furthermore, the drug should also have enough specificity to compete and interact exclusively with its target minimizing its potential interaction with thousands of other intracellular compounds. The most used method to study protein–protein interactions in cells is the yeast two-hybrid system (Y2H) (ref. 1 ). This method has a clear advantage over classical in vitro biochemical approaches such as co-(immuno)precipitation and co-purification analyses, as it embodies an in vivo technique using the yeast host cell as a live test tube. The Y2H is based on the activation of the expression of a downstream reporter gene mediated by the binding between two proteins of interest. Ultimately, this gene expression drives a change in yeast cell’s phenotype that can be indirectly linked back to the interaction between the proteins under study. This method has been widely used because of its high-throughput screening capability and powerful ability to identify unknown protein-binding partners. A natural obstacle is that the two-hybrid system makes use of the yeast Sacharomyces cerevisiae as a host and uses a specific reporter gene. This imposes limitations upon interactions specific to mammalian pathways that do not occur in yeast and/or do not take place in the (yeast) cell nucleus. Furthermore, it relies on activation of gene expression and, as a consequence, cannot be used with proteins that are self-activating by themselves. Several fluorescent techniques such as FRET/FLIM have been developed during the last years as alternatives to study protein–protein interactions [2] , [3] . These methods require specialized equipment, special fluorophore combinations, specific acquisition software tools and/or complex post acquisition data analysis. Here we propose a simple and general method that can be applied and adapted to study protein interactions in any species, cell type and intracellular compartment. A major advantage is that this technology does not depend on the activation of any specific reporter gene and the interaction between proteins can be studied in real time at any location within a live cell. This strategy is based on a high-affinity anti-GFP nanobody. This anti-GFP nanobody was screened and optimized to reach an affinity to GFP in the subnanoMolar range [4] . The basic rationale of the method is shown in Fig. 1a . A protein with high affinity to GFP (GFP-binding nanobody), which we call GFP binder protein (GBP), is covalently linked to a protein that accumulates at a specific location within the cell. We call these fusions between GBP and a localization protein (LP) GBP–LP. In this way, a GFP-labelled protein is artificially recruited to a specific location. Using a different fluorescent label for the second protein of interest then allows easy detection and measurement of the interaction between the two proteins (hence fluorescence three-hybrid assay—F3H). A convenient aspect of this method is that, after the GBP–LP plasmid is constructed, the same intracellular location determined by the LP can be used to study the interaction between any numbers of proteins where one of them is labelled with GFP. 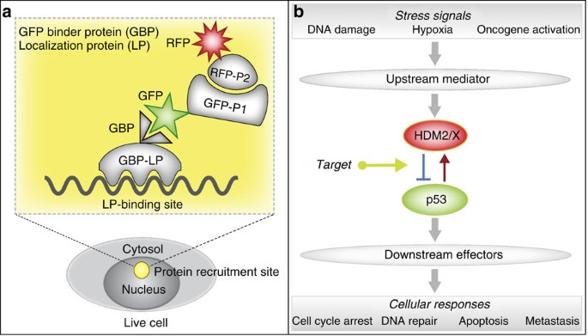Figure 1: Strategy for visualizing protein interactions in living cells and outline of a fundamental biological application. (a) Schematic representation of the fluorescence three-hybrid (F3H) to study protein–protein interactions. A GFP binder protein (GBP) is attached to a protein (LP) that accumulates at a well-defined location within the cell. This complex recruits to that particular location GFP-tagged proteins (GFP-P1). If the protein P1 interacts with a second protein P2, labelled with a different fluorescent marker, the interaction can be immediately visualized using fluorescent microscopy. (b) Schematic representation of the interaction between p53 and HDM2/X and its central role in cellular regulation and genome preservation. Figure 1: Strategy for visualizing protein interactions in living cells and outline of a fundamental biological application. ( a ) Schematic representation of the fluorescence three-hybrid (F3H) to study protein–protein interactions. A GFP binder protein (GBP) is attached to a protein (LP) that accumulates at a well-defined location within the cell. This complex recruits to that particular location GFP-tagged proteins (GFP-P1). If the protein P1 interacts with a second protein P2, labelled with a different fluorescent marker, the interaction can be immediately visualized using fluorescent microscopy. ( b ) Schematic representation of the interaction between p53 and HDM2/X and its central role in cellular regulation and genome preservation. Full size image To establish and validate the basis of this strategy, we focused on the binding and disruption of p53 and HDM2 (human double minute 2) as this is one of the most important protein interactions in cancer research. The tumour suppressor p53, also named the ‘guardian of the genome’, is the main mediator of apoptosis, cell cycle arrest and senescence in response to a broad range of DNA damages and other cellular stresses ( Fig. 1b ). Depending on the stress signal, p53 gets modified and activated by upstream mediators that lead p53 to activate diverse genes and response pathways. The induction of high levels of p53 prevents inappropriate propagation of mutant cells. The intracellular p53 level is the single most important determinant of its function and HDM2 is the principal cellular antagonist of p53, blocking its tumour suppressor function by binding to its transcription activation domain. The two proteins bind to each other as part of a negative autoregulatory loop aimed to keep low p53 levels in the absence of stress. HDM2 blocks p53 by binding to its transcription domain and reduces its levels acting as an E3 ubiquitin ligase polyubiquitinating p53 and targeting it for degradation [5] , [6] . In all cancers, the functions of p53 are limited allowing these cells to evade apoptosis and cell growth arrest [7] . About half of all cancers retain wild-type fully functional p53 (ref. 8 ) and in these the normal regulation of p53 is in many cases disrupted through direct overexpression of HDM2 [9] . Overexpression of HDM2 provides a growth advantage to cells, promotes tumorigenesis and correlates with very poor response to cancer therapy and consequently bad prognosis [9] , [10] , [11] , [12] . Simultaneous mutation of p53 and amplification of HDM2 does not generally occur within the same tumour, suggesting that HDM2 amplification is an effective way to block p53 function [9] , [13] , [14] . We present a simple visualization method for immediate recognition of protein–protein interactions, which represents a first step in capturing the kinetics of protein–protein interaction and for high-throughput methods. These types of studies are central to expand our mechanistic understanding of drug function in vivo . Visualizing and quantifying interactions in live cells The F3H assay offers the opportunity to determine whether the proteins are interacting from a single-fluorescence snapshot as shown in Fig. 2 . To visualize the interaction between p53 and HDM2, we coupled the GBP to the Lac repressor (LacI). In cell lines where an array composed of Lac operator DNA sequence repeats has been stably integrated in the genome, such as in baby hamster kidney (BHK) cells [15] , the GBP–LacI binds to the Lac operator array ( LacO ). This recruits GFP-labelled proteins to the LacO region within the nucleus. If a second protein labelled with a different fluorescent molecule interacts with the GFP-labelled protein, then it will also display an accumulation at the LacO region. As shown in Fig. 2 without tethering to a particular location the difference in correlation between images (a) and (b) is very weak and the interaction or lack thereof would be difficult to score. Using the GBP–LacI sharply enhances the correlation contrast between interacting and non-interacting proteins. This can be used to determine in single snapshots the interaction between proteins of interest. This fast and efficient visualization strategy allows following in real time the dynamics of intracellular processes and the effects of inhibitors. 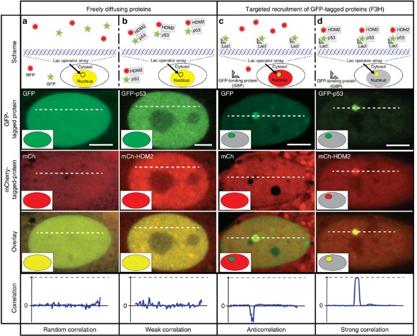Figure 2: Targeted recruitment of GFP-tagged proteins allows visualization and quantification of protein–protein interactions in live cells. Re-localization of GFP-tagged proteins (tethered; immobilized; recruited) to theLacoperator using the GBP–LacI. Confocal microscopy images of non-interacting GFP and mCherry are shown and interacting GFP–p53 (pNeG-p53(NTD)) and mCh–HDM2 (pCAG-Ch-HDM2(NTD)) proteins in live cells co-transfected with and without the GBP–LacI. In the first row, a schematic representation of the transfected constructs and the respective protein distribution is shown, in the second row, a confocal image of the GFP-tagged protein, in the third row, an image of the mCherry-tagged protein, in the fourth row, the overlay of the two previous channels and in the last row, the derivative of the Pearson’s correlation coefficient between the GFP image and the mCherry image along the dotted line drawn in the confocal images. In columns (a–d) representative images of cells transiently transfected with the constructs indicated in the respective schemes above are shown. Scale bar, 5 μm. Figure 2: Targeted recruitment of GFP-tagged proteins allows visualization and quantification of protein–protein interactions in live cells. Re-localization of GFP-tagged proteins (tethered; immobilized; recruited) to the Lac operator using the GBP–LacI. Confocal microscopy images of non-interacting GFP and mCherry are shown and interacting GFP–p53 (pNeG-p53(NTD)) and mCh–HDM2 (pCAG-Ch-HDM2(NTD)) proteins in live cells co-transfected with and without the GBP–LacI. In the first row, a schematic representation of the transfected constructs and the respective protein distribution is shown, in the second row, a confocal image of the GFP-tagged protein, in the third row, an image of the mCherry-tagged protein, in the fourth row, the overlay of the two previous channels and in the last row, the derivative of the Pearson’s correlation coefficient between the GFP image and the mCherry image along the dotted line drawn in the confocal images. In columns ( a – d ) representative images of cells transiently transfected with the constructs indicated in the respective schemes above are shown. Scale bar, 5 μm. Full size image Inhibition kinetics of p53–HDM2 binding induced by Nutlin 3 The realization that HDM2 is the master regulator of p53 has triggered the idea of developing an inhibitor for this interaction. From a broader perspective, this is one of the first examples in which it has been clearly shown that protein–protein interactions can be efficiently disrupted by small molecule inhibitors. It was long believed that protein–protein interactions could not be effectively inhibited with small molecules because of the large and poor definition of protein interfaces [16] . This view has recently changed and targeting the interaction between HDM2 and p53 using small molecular compounds in tumour cells has become a primary therapeutic strategy. Consequently, a large number of small chemical compounds are currently being screened and engineered. Among them, the Nutlins [17] are the most studied. The Nutlins are the first examples of potent and specific inhibitors of the HDM2–p53 interaction and one of them, Nutlin 3, has been extensively evaluated for its therapeutic potential and mechanism of action in human cancer. A key advantage of the method proposed here is that it allows in live cells an immediate determination of the interaction between any pair of proteins in which one of them is labelled with GFP. This means that with a single-fluorescence snapshot at a given time point it makes it possible to determine the interaction relative to a previous time point. This allows resolving fast kinetics in live cells such as the inhibition of these interactions after treatment with a given drug. To test this approach, we measured in live cells the disruption kinetics of the p53 and HDM2 interaction upon treatment with Nutlin 3 ( Fig. 3 , Supplementary Fig. S1 ). BHK cells (containing a stably integrated LacO DNA array) were transiently transfected with constructs coding for GBP–LacI, GFP–p53 and mCh–HDM2. GFP–p53 gets bound to the LacO array by its interaction with GBP–LacI. Before the treatment with Nutlin 3, HDM2 labelled with mCherry is also recruited to the LacO by its interaction with p53. No unspecific binding of p53, HDM2, GFP or mCherry to the LacO was detected ( Supplementary Fig. S2 ). 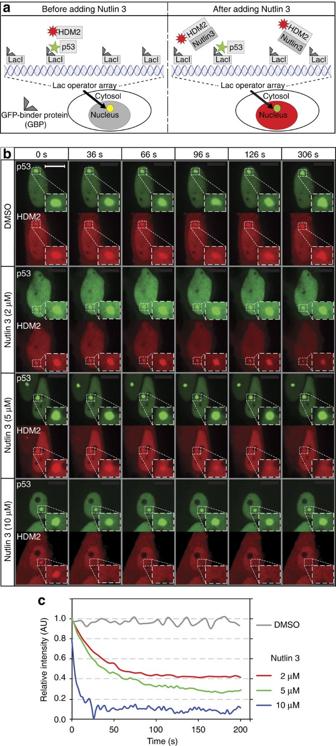Figure 3: Visualization of targeted disruption of protein interactions in live cells. BHK cells containing a stably integratedLacOarray were transiently transfected with pNeG-p53(NTD), pCAG-Ch-HDM2(NTD) and GBP–LacI. In (a) is shown a schematic representation of the re-localization of the GFP–p53 to theLacOarray, its interaction with mCh–HDM2 and the disruption of this interaction mediated by Nutlin 3. (b) Live cell confocal microscopy images showing the disruption kinetics of the interaction between HDM2 and p53 mediated by Nutlin 3 at 0 (DMSO, control), 2, 5 and 10 μM. (c) Time lapse quantification of the relative binding of p53 to HDM2. Higher concentrations of Nutlin 3 resulted in faster disruption of the interaction between the proteins. InSupplementary Fig. S1are shown the kinetic traces, the mean and the s.e. of the interaction disruption mediated by Nutlin 3 at 5 μM obtained from five repetitions showing the reproducibility of the individual traces. Scale bar, 5 μm. Figure 3a shows a cartoon representation of the interactions and signals before and after the treatment with Nutlin 3. Figure 3b shows the fluorescent images of the cells for each protein at different concentrations of Nutlin 3 and different time points. In Fig. 3c , the intensity ratio of mCh–HDM2 at the LacO after the treatment with Nutlin 3 is plotted relative to its intensity before the drug treatment. We observed that the time scale of the disruption is within seconds after treatment with Nutlin 3. This disruption can be partial at concentrations below 10 μM and is almost complete at 10 μM. As mentioned previously, it was already surprising a few years ago that small molecules can disrupt the binding of proteins. We can now in addition directly measure the fast disruption kinetics of these interactions in live mammalian cells. Furthermore, with this assay we obtained accurate and reproducible results over a broad range of expression ratios as shown in the automated analysis in Supplementary Fig. S3 . Figure 3: Visualization of targeted disruption of protein interactions in live cells. BHK cells containing a stably integrated LacO array were transiently transfected with pNeG-p53(NTD), pCAG-Ch-HDM2(NTD) and GBP–LacI. In ( a ) is shown a schematic representation of the re-localization of the GFP–p53 to the LacO array, its interaction with mCh–HDM2 and the disruption of this interaction mediated by Nutlin 3. ( b ) Live cell confocal microscopy images showing the disruption kinetics of the interaction between HDM2 and p53 mediated by Nutlin 3 at 0 (DMSO, control), 2, 5 and 10 μM. ( c ) Time lapse quantification of the relative binding of p53 to HDM2. Higher concentrations of Nutlin 3 resulted in faster disruption of the interaction between the proteins. In Supplementary Fig. S1 are shown the kinetic traces, the mean and the s.e. of the interaction disruption mediated by Nutlin 3 at 5 μM obtained from five repetitions showing the reproducibility of the individual traces. Scale bar, 5 μm. Full size image High-throughput analysis of interaction disruption by drugs A clear visualization technology for these interactions can be used to develop efficient methods for high-throughput screening. Therefore, in Supplementary Fig. S4 we outline this idea comparing Nutlin 3 with other well-studied chemical compounds. In particular, we compared the effect of three drugs, RITA, Nutlin 3 and Mi 63. Using Nutlin 3 as reference and DMSO as a control, we observed that Mi 63 displays a stronger inhibition than Nutlin 3, while RITA does not disrupt the p53–HDM2 interaction. It has been shown that RITA has antitumor effects and it was originally proposed that it does so by disrupting the p53–HDM2 (ref. 18 ). In vitro NMR studies [19] have contested this suggesting that RITA does not disrupt p53–HDM2 interaction. Our results, now in live mammalian cells, agree and extend the in vitro NMR analysis. Design of a cell-permeable peptide inhibitor Several very strong peptide inhibitors have been reported [20] besides small chemical compounds like the Nutlins. Some of these peptides have been optimized to display a double high affinity not only for HDM2 but also for HDMX [20] . Using phage display peptide libraries a potent dual peptide inhibitor for HDM2 and HDMX, here named N8A, has been reported [21] ( Fig. 4a ). In vitro , this peptide has several fold higher binding affinity for HDM2 than the corresponding p53-binding region [21] . 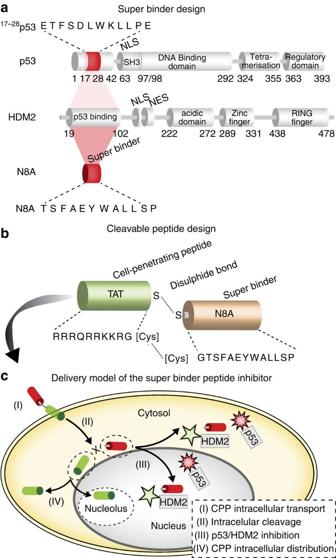Figure 4: Rationally designedin vivocleavable cell-permeable peptide to inhibit and disrupt the binding between p53 and HDM2. (a) Short sequence from p53 responsible for the binding between p53 and HDM2. Below this sequence the main domains of p53 and HDM2 are depicted along with a short peptide (N8A) that has been shownin vitroto have higher affinity for HDM2 than p53. (b) The N8A peptide is not able to reach the interior of living cells. Therefore, it was coupled by a disulphide bond to a cell-penetrating peptide (TAT) that is capable of transporting it into living cells. (c) The design is based on a delivery model in which (I) the TAT peptide transports the N8A peptide into the cell, (II) in the cytosol the disulphide bridge is cleaved releasing the N8A peptide from the TAT peptide, (III) the peptide inhibitor is free to diffuse throughout the nucleus and the cytosol inhibiting the binding between p53 and HDM2, (IV) while the TAT peptide accumulates preferentially at the cytosol and the nucleolus. Figure 4: Rationally designed in vivo cleavable cell-permeable peptide to inhibit and disrupt the binding between p53 and HDM2. ( a ) Short sequence from p53 responsible for the binding between p53 and HDM2. Below this sequence the main domains of p53 and HDM2 are depicted along with a short peptide (N8A) that has been shown in vitro to have higher affinity for HDM2 than p53. ( b ) The N8A peptide is not able to reach the interior of living cells. Therefore, it was coupled by a disulphide bond to a cell-penetrating peptide (TAT) that is capable of transporting it into living cells. ( c ) The design is based on a delivery model in which (I) the TAT peptide transports the N8A peptide into the cell, (II) in the cytosol the disulphide bridge is cleaved releasing the N8A peptide from the TAT peptide, (III) the peptide inhibitor is free to diffuse throughout the nucleus and the cytosol inhibiting the binding between p53 and HDM2, (IV) while the TAT peptide accumulates preferentially at the cytosol and the nucleolus. Full size image Small chemical compounds such as the Nutlins do not show inhibition of the p53–HDMX interaction [22] . Therefore, these peptides offer a clear advantage. However, they lack cell permeability, which is essential for targeting these intracellular proteins in vivo . To solve this issue, as shown schematically in Fig. 4b , we coupled this peptide inhibitor to cell-penetrating peptides (CPPs) [23] , [24] , [25] , [26] , [27] . CPPs are short basic peptides, ~10 amino acids, capable of crossing the cell plasma membrane transporting other covalently attached molecules such as peptides avoiding endosomal trapping and degradation [26] . Using CPPs to deliver these small inhibitors has the potential disadvantage that the CPP itself can interfere with the binding of the inhibitor to the target. To overcome this potential issue, as shown in Fig. 4c , we coupled the peptide inhibitor to the CPP, in this case the TAT peptide, using a disulphide bridge so that once in the cytosol, the disulphide bridge is reduced and the inhibitor peptide is released becoming free to target HDM2. Visualization at different subcellular locations An important aspect of the F3H strategy is that it can be used with any cell type. In Fig. 5a and Supplementary Movie 1 we made use of the re-localization of GFP-tagged proteins to the LacO DNA array, for which it is required to have first the DNA array permanently incorporated into the cell’s genome. However, with the F3H we can now use other existing structures within the cells. In the next step, we expanded the system to any mouse cell taking advantage of the naturally occurring major satellite DNA repeats rich in methylated cytosines at pericentric regions of each and every mouse chromosome. To this purpose, we made use of a fusion of the GBP with the methyl cytosine-binding domain (MBD) of MeCP2, which is known to accumulate at these chromosomal domains, also called chromocenters in interphase cells [28] , [29] . The outcome is shown in Fig. 5b where both p53 and HDM2 initially could be seen colocalizing at chromocenters and upon peptide addition total disruption of the interaction can be scored by the re-localization of the p53 away from these structures. To make the system extendable to any cell containing lamina, and not only any mouse cells, we fused the GBP to lamin B1. In this way, we could target the GFP-fusion protein to the nuclear periphery, using, for example, human HeLa cells and assay for the release of the interacting protein from the lamina. The outcome in human cells is shown in Fig. 5c and upon disruption by the addition of the peptide, the red-labelled p53 protein is seen only in the nucleoplasm displaced from the nuclear periphery. In Supplementary Fig. S5 is shown the automated detection and analysis of protein–protein interactions at the nuclear lamina using a high-throughput wide-field microscopy system. Finally, to test whether the assay would work also in the cytosol we fused the GBP to centrin and, hence targeted the GFP-fusion to the centrioles. As shown in Fig. 5d , the colocalization and, upon peptide addition, disruption of the p53 and HDM2 interaction could also be easily measured in the cytosol. In Supplementary Fig. S6 is shown the automated detection and analysis of protein–protein interactions at the centrioles using a high-throughput system. Thus, our approach is totally flexible and is applicable to various subcellular compartments, cell types and species. 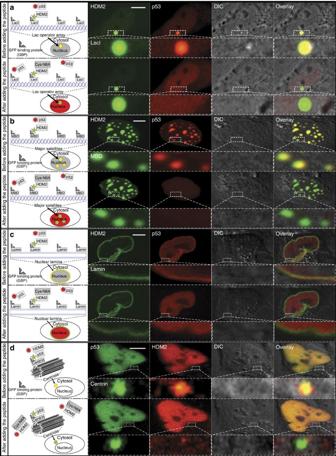Figure 5: A rationally designedin vivocleavable cell-permeable peptide that inhibits and disrupts the binding between p53 and HDM2. The peptide was tested in several mammalian cell lines (a–d). Starting from hamster cell lines containing stably integrated Lac operator (LacO) DNA arrays, the system is expanded onto application on any mouse cell exploiting the natural occurrence of large regions around centromeres naturally containing arrays of major satellite DNA sequences rich in methylated cytosines and, hence, accumulating methyl cytosine-binding domain (MBD) proteins. On a next step, the system is expanded to any cell containing a nuclear lamina composed of lamin intermediate filament proteins. Finally, the system is transferred to the cytosol making use of targeting it to the centrioleviathe centrin protein. In the first column, a cartoon representation of the protein interactions and inhibition at each recruitment site within the cell is shown. In the second column, a confocal image of a representative live cell of the GFP channel is shown followed by the mCherry channel in the third column, a transmission light image in the fourth column and in the last column the overlay of all the channels. In each row are shown the images before and after adding the N8A peptide to a final concentration of 8 μM. An amplified image of the recruitment site is shown below each microscopic image. (a) Recruitment of GFP-HDM2 to theLacOarray in hamster BHK cells. Cells transiently transfected with pNeG-HDM2(NTD), pCAG-Ch-p53(NTD) and GBP–LacI. (b) Recruitment of GFP-HDM2 to major satellite pericentric repeats rich in MBD proteins in mouse C2C12 cells. Cells transiently transfected with pNeG-HDM2(NTD), pCAG-Ch-p53(NTD) and GBP-MBD (c) Recruitment of GFP-HDM2 to the nuclear lamina in human HeLa cells. Cells transiently transfected with pNeG-HDM2(NTD), pCAG-Ch-p53(NTD) and GBP-Lamin B1. (d) Recruitment of p53-GFP to the centriole in HeLa cells. Cells transiently transfected with p53-GFP, pCAG-Ch-HDM2(NTD) and GBP-Centrin2. Scale bar, 5 μm. Figure 5: A rationally designed in vivo cleavable cell-permeable peptide that inhibits and disrupts the binding between p53 and HDM2. The peptide was tested in several mammalian cell lines ( a – d ). Starting from hamster cell lines containing stably integrated Lac operator ( LacO ) DNA arrays, the system is expanded onto application on any mouse cell exploiting the natural occurrence of large regions around centromeres naturally containing arrays of major satellite DNA sequences rich in methylated cytosines and, hence, accumulating methyl cytosine-binding domain (MBD) proteins. On a next step, the system is expanded to any cell containing a nuclear lamina composed of lamin intermediate filament proteins. Finally, the system is transferred to the cytosol making use of targeting it to the centriole via the centrin protein. In the first column, a cartoon representation of the protein interactions and inhibition at each recruitment site within the cell is shown. In the second column, a confocal image of a representative live cell of the GFP channel is shown followed by the mCherry channel in the third column, a transmission light image in the fourth column and in the last column the overlay of all the channels. In each row are shown the images before and after adding the N8A peptide to a final concentration of 8 μM. An amplified image of the recruitment site is shown below each microscopic image. ( a ) Recruitment of GFP-HDM2 to the LacO array in hamster BHK cells. Cells transiently transfected with pNeG-HDM2(NTD), pCAG-Ch-p53(NTD) and GBP–LacI. ( b ) Recruitment of GFP-HDM2 to major satellite pericentric repeats rich in MBD proteins in mouse C2C12 cells. Cells transiently transfected with pNeG-HDM2(NTD), pCAG-Ch-p53(NTD) and GBP-MBD ( c ) Recruitment of GFP-HDM2 to the nuclear lamina in human HeLa cells. Cells transiently transfected with pNeG-HDM2(NTD), pCAG-Ch-p53(NTD) and GBP-Lamin B1. ( d ) Recruitment of p53-GFP to the centriole in HeLa cells. Cells transiently transfected with p53-GFP, pCAG-Ch-HDM2(NTD) and GBP-Centrin2. Scale bar, 5 μm. Full size image In summary, the cell-based method presented here can be used to study protein–protein interactions and their inhibition in vivo in any cell type. In particular, it provides real-time kinetics of these interactions in live cells and can be applied to characterize and/or screen for specific inhibitors. We applied and validated the F3H approach by visualizing the binding and targeted disruption of p53 and HDM2 in real time in live cells using different drugs including Nutlin 3 and a novel cell-permeable and in vivo cleavable peptide inhibitor. Peptide synthesis and analyses The individual peptides were synthesized by BIOSYNTAN GmbH using simultaneous peptide synthesis on the following instruments: SYRO, MultiSynTec GmbH, Germany, using the Fmoc/But strategy developed Sheppard. Couplings were performed using 3–6 equiv Fmoc-amino acid/HOBt/TBTU and 6–12 equiv N -methylmorpholine in the following resin: Tentagel HL RAM resin; RAPP Polymere GmbH, Tuebingen, Germany, loading 0.36 mmol g −1 resin. The peptide fragment RRRQRRKRGC was synthesized with dipyridyl-disulphide during the deprotection reaction. The unsymmetrical dimerization between the TAT peptide fragment RRRQRRKRGC and the N8A peptide CGTSFAEYWALLSP-amide ( Supplementary Fig. S7 ) was performed in solution (pH 6.0). The protecting groups used are: Cys(Trt), Arg(Pbf), Ser(But), Thr(But), Tyr(But), Asp(OBut), Glu(OBut), Asn(Trt), Gln(Trt), Lys(Boc), His(Trt) and Trp(Boc). Peptides were deprotected and cleaved from the resin by trifluoroacetic acid (TFA)/water (95:2.5) 2 h, room temperature; adding 3% triisopropylsilane [30] . For preparative HPLC, the HPLC instrument Shimadzu LC-8A with UV–vis detector SPD-6A was used with an Ultrasep ES (RP-18), 10 μm, (250 × 20 mm) column. Solvent was as described below with a corresponding gradient in 30 min. Flow: 15.0 ml min −1 . Detection: 220 nm. For analytical HPLC, the HPLC Shimadzu LC-9A with photodiode array detector SPD-M6A was used with an Ultrasep ES (RP-18), 7 μm, (250 × 3.0 mm) column. Solvent A=0.05% TFA in water; solvent B=0.05% TFA in 80% ACN/water. Flow: 0.6 ml min −1 . Linear gradient: 2.5% B per min. Detection: 220 nm ( Supplementary Fig. S8 ). Peptides were further analysed by MALDI-TOF using a MALDI2 DE instrument, Shimadzu, Japan, in linear mode. Calculated molecular weight as average mass: 3,040.6; molecular weight detected: 3,041.4 ( Supplementary Fig. S9 ). Plasmids The mammalian expression constructs coding for HDM2 and p53 deletions as well as p53 full-length protein fused with eGFP or mCherry are schematically shown in Supplementary Fig. S10 together with the GFP binder nanobody [31] , [32] (GBP)-localization constructs used to recruit the GFP-tagged proteins to different regions within the cell. The DNA sequence coding for the N-terminal domain of p53 (aa 1–81) and HDM2 (aa 1–128) were amplified from human cDNA by PCR using fusion high-fidelity DNA Polymerase (New England BioLabs) and cloned in frame into NLS-eGFP, or eGFP, or mCherry plasmids with Asi SI and Not I restriction endonucleases (New England BioLabs). The human full-length p53 fused to GFP was obtained from Addgene (catalogue no. 12091) [33] . pGBP-LacI was constructed by deleting the mRFP-coding sequence from pGFPbinderImR plasmid using Bam HI and Bsr GI restriction endonucleases [34] . GBP-LaminB1 was described previously [31] . To construct the pMBD-GBP plasmid, pEGFP-C2 vector (CLONTECH Laboratories, Inc.) was digested by Nhe I and Hind III (New England BioLabs), and the MBD domain of rat MeCP2 and GBP were both ligated into the backbone. pGBP-Centrin was constructed by replacing the LacI of pGBP-LacI with the Centrin2 ORF using Bam HI and Hind III restriction endonucleases (New England BioLabs). Cell culture and transfection The following cell lines were used in this study: BHK cells containing multiple lac operator [15] repeats, C2C12 mouse myoblast cells [35] , U2OS human osteosarcoma cells [36] , HeLa human cervical carcinoma cells [37] . All cell lines where grown in a humidified atmosphere at 37 °C and 5% CO 2 , in Dulbecco’s modified Eagle’s medium (DMEM) supplemented with 1 μM gentamycin and 10% (BHK, U2OS and HeLa) or 20% (C2C12) fetal calf serum. All cell lines were transiently transfected using PEI (poly-ethyleneimine; 1 mg ml −1 in ddH 2 O, neutralized with HCl). For the transfection, 200 μl DMEM serum-free with 12 μl of PEI was vortexed for 2 min and added to 200 μl serum-free DMEM with 4 μg DNA. After incubating the DNA-PEI mixture for 15 min at room temperature, the solution was added to the cells drop wise and incubated overnight at 37 °C and 5% CO 2 . Drug treatment Nutlin 3 (Sigma) was dissolved in DMSO as a 10 mM stock solution. Mi 63 and RITA were a kind gift from Dr. Holak (MPI Biochemistry, Martinsried, Germany). For high-throughput assays BHK cells plated onto 96-well plates (Greiner Bio-One) were triple-transfected with the plasmids indicated in the corresponding figures. Sixteen hours later, the medium was changed to phenol red free medium supplemented with the Nutlin 3 or the other compounds at various concentrations for 30 min, then fixed with 3.7% formaldehyde and DNA counterstained with DAPI. For each concentration, triplicate wells were treated. For live cell microscopy cells were plated on poly- L -Lysine coated eight-well μ-Slide (ibidi GmbH) and transfected as described. Cells were imaged live on a spinning disk confocal system before and immediately after addition of Nutlin 3 or peptide inhibitors. High-throughput microscopy and image analysis After cell fixation, images were acquired automatically with an Operetta high-content imaging system at the wide-field mode using a × 40 air objective (PerkinElmer). DAPI, eGFP and Cherry fluorescent fusion proteins were excited and the emissions were recorded using standard filter sets. Exposure time was controlled to avoid saturated pixels, typically from 50–200 ms, 30 different fields were imaged in each well. The imaging time can be calculated as 150 ms per channel × 3 channels × 30 fields per well × 96 wells=1,296 s=21.6 min, adding to this the time for objective movement, refocusing, filter swapping, the total time for 96-well plate takes about 90 min. The images were then analysed with the Harmony analysis software (PerkinElmer) with a flow diagram shown in Supplementary Fig. S11 . Briefly, the images were first segmented by intensity and area size according to the DAPI fluorescence using the top-hat method to define the cell nucleus area (cells, blue in Supplementary Fig. S11 ), and nucleus masks were produced and recorded. Then the LacO foci were recognized by intensity in the eGFP channel within the nucleus areas, which were defined in the former step, and cells with one LacO spot were kept for subsequent analysis (cells with spot, green in Supplementary Fig. S11 ). The cell with one green spot in the nucleus and a red signal was considered as triple-transfected cell with a spot (brown in Supplementary Fig. S11 ). In these cells, the mean intensities of mCherry channel at the LacO were recorded according to LacO foci masks gotten from the GFP channel, and the ratio of mCherry mean intensity at the LacO spot (spot mCherry ) to the mean intensity of whole nucleus (nucleus mCherry ) were calculated, and then used to subgroup the cells into ‘interacting cells’ (yellow in Supplementary Fig. S11 ) or ‘non-interacting cells’. The percentages of ‘interacting cells’ in each well were plotted and used as an indication of the drug inhibitory effect. Depending on the application, it might be helpful to also consider the relative enrichment of mCherry fusion proteins at the LacO . Live cell confocal microscopy and image analysis Transfected cells plated on μ-Slide 8-well were selected and imaged in peptide inhibitor-free medium. Immediately after addition of the peptide inhibitor at 8 μM final concentration, 3D stacks were acquired at 1 min time intervals for up to 1 h. Time lapse imaging was carried out on a UltraVIEW VoX spinning disc confocal system (PerkinElmer, UK) in a closed live cell microscopy chamber (ACU control, Olympus, Japan) heated to 37 °C, with 5% CO 2 and 60% air humidity, mounted on a Nikon Ti microscope (Nikon, Japan). Image acquisition was performed using a × 60/1.45 NA Planapochromat oil immersion objective lens. Images were obtained with a cooled 14-bit EMCCD camera (C9100-50, CamLink). To visualize the GFP signal, a 488 nm excitation laser and a 521-nm emission filter were used, the mCherry protein was excited using a 561-nm laser and the emission was filtered through a 587 nm filter. For the analysis of correlation between fluorescent signals in Fig. 2 , the derivative of the Pearson’s coefficient along the plotted line was computed. This shows the change in correlation along the selected line. The intensity plot in Supplementary Movie 1 was computed by extracting first the LacI spot, at each z-stack confocal plane, by computing the mean GFP intensity over the nucleus and extracting the pixels with intensity values 1.5 times higher than the mean. We visually verified that these criteria were correctly extracting only the LacI spot. After extracting the LacI spot for each confocal plane of the z-stack, this was used as a mask to extract the pixels corresponding the LacI spot in the mCherry channel. The GFP and mCherry signals at the LacI spot were normalized by dividing the intensity in each pixel by the average intensity of each signal in the nucleus. The plot shows the result after the integration of these normalized signals at the LacI spot before and after adding the peptide inhibitor. To perform this analysis, we wrote a program that performed automatically this analysis at each time point, and produced as an output the plot and the movie. How to cite this article: Herce, H. D. et al. Visualization and targeted disruption of protein interactions in living cells. Nat. Commun. 4:2660 doi: 10.1038/ncomms3660 (2013).